Tailoring the chirality of magnetic domain walls by interface engineering Contacting ferromagnetic films with normal metals changes how magnetic textures respond to electric currents, enabling surprisingly fast domain wall motions and spin texture-dependent propagation direction. These effects are attributed to domain wall chirality induced by the Dzyaloshinskii–Moriya interaction at interfaces, which suggests rich possibilities to influence domain wall dynamics if the Dzyaloshinskii–Moriya interaction can be adjusted. Chiral magnetism was seen in several film structures on appropriately chosen substrates where interfacial spin-orbit-coupling effects are strong. Here we use real-space imaging to visualize chiral domain walls in cobalt/nickel multilayers in contact with platinum and iridium. We show that the Dzyaloshinskii–Moriya interaction can be adjusted to stabilize either left-handed or right-handed Néel walls, or non-chiral Bloch walls by adjusting an interfacial spacer layer between the multilayers and the substrate. Our findings introduce domain wall chirality as a new degree of freedom, which may open up new opportunities for spintronics device designs. Formation and structure of domain walls (DWs) is usually thought to result from the interplay between exchange interaction, magnetic anisotropy and dipolar interaction, and Bloch walls are predicted as the lowest energy walls in perpendicularly magnetized systems [1] , [2] , [3] . Crossing a Bloch wall, the spin vector rotates like a spiral and, in this picture, right-handed and left-handed rotating DWs are thought to be degenerate as a result of the symmetric exchange interaction. The absence of inversion symmetry at surfaces or interfaces breaks the inversion invariance of the symmetric exchange interaction in the presence of spin-orbit coupling; this introduces a Dzyaloshinskii–Moriya interaction (DMI) term into the free energy of the system, which can lift the left/right degeneracy [4] , [5] . The DMI term can be written as E DM = D ij ·( S i × S j ), where D ij is the DMI vector, and S i and S j are magnetic spin moments located on neighbouring atomic sites i and j . With a sufficiently strong DMI, the ground state of DWs in perpendicularly magnetized systems evolves into a homochiral Néel wall structure [6] , [7] , where the spin vector rotates like a cycloid across the DW. In magnetic films that are in contact with normal metals, experimental examination of current-driven DW dynamics in the presence of external magnetic field indicated DW chirality [8] , [9] . These reports showed that DW chirality can explain observations of surprisingly fast DW motions and even the possibility of reversed propagation direction [8] , [9] , [10] . In addition, recent theoretical results suggest rich possibilities to influence DW dynamics if the DMI can be manipulated [6] , [11] , [12] . In thin film systems grown on appropriately chosen substrates where interfacial spin-orbit-coupling effects are strong, magnetic chiral order was seen in the spin structure of DWs [7] , in magnetic cycloids [13] , [14] , [15] and in skyrmion structures [16] . The goal of our present work is to directly visualize the extent of DW chirality in magnetic thin films in contact with normal metal. Moreover, we aim to develop an experimental foundation for manipulating the strength and sign of the DMI and magnetic chirality. We chose to investigate [Co/Ni] n multilayers, which is a prototypical perpendicularly magnetized system [17] , [18] , and it is an important model for studies of current-induced DW motion [19] , [20] , [21] , [22] for future logic and memory devices [23] , [24] and current-driven magnetization reversal in nanopillars [25] for data storage [26] . However, experimental measurements directly revealing the spin structure of DWs in this system are still missing. Here we image chiral DWs in [Co/Ni] n multilayers in contact with Pt and Ir by using spin-polarized low-energy electron microscopy (SPLEEM) [27] , [28] , [29] . We show that by adjusting the thickness on an Ir spacer layer between [Co/Ni] n multilayers and a Pt substrate, the DMI can be manipulated to stabilize either left-handed or right-handed Néel walls or non-chiral Bloch walls. Our findings provide firm experimental evidence for the presence of homochiral spin texture and introduce DW chirality as a new degree of freedom that can be controlled through interface engineering, which may open up new opportunities for spintronics device designs [23] , [24] . 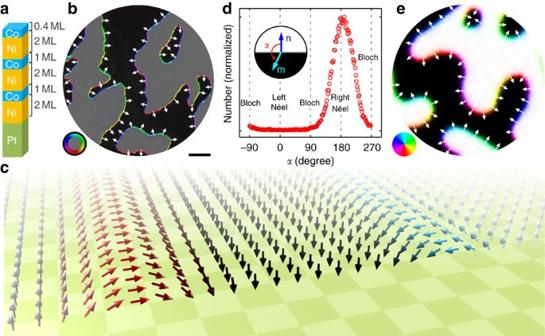Figure 1: Real-space observation of chiral Néel walls in [Co/Ni]nmultilayer. (a) Sketch of [Co/Ni]3grown on Pt(111) substrate. (b) Compound SPLEEM images highlighting the DW. The colour wheel represents the direction of in-plane magnetization in each image pixel. White arrows show the in-plane spin orientations in the DWs. Scale bar, 2 μm. (c) Sketch of right-handed Néel wall. (d) Histogram of angleαin DW boundary counted pixel-by-pixel inbshows a Gaussian distribution peaked at 180°, which corresponds to right-handed Néel wall. Inset shows the definition of the angleα, wherenis a unit vector perpendicular to the domain boundary and always points from black domain to grey domain,mis the in-plane direction of the magnetization within the DW. (e) Monte Carlo simulation result of perpendicular magnetized film with the DMI shows right-handed chiral Néel walls with similar spin structures as seen experimentally inb. Visualizing chiral DWs Figure 1 shows a SPLEEM measurement of the DW spin structure in a [Co/Ni] n multilayer stack epitaxially grown on Pt(111) (structure of the stack sketched in Fig. 1a ). In the compound SPLEEM image reproduced in Fig. 1b , in-plane components of DWs are highlighted in colour as indicated by a colour wheel (inset), and the perpendicular magnetization component is shown by black and grey. The magnetization within DWs always points from grey domains (+ M z ) to black domains (− M z ), independent of the direction of the domain boundary (see white arrows in Fig. 1b ). This spin structure corresponds to right-handed chiral Néel walls [7] , [30] as sketched in Fig. 1c . Figure 1: Real-space observation of chiral Néel walls in [Co/Ni] n multilayer. ( a ) Sketch of [Co/Ni] 3 grown on Pt(111) substrate. ( b ) Compound SPLEEM images highlighting the DW. The colour wheel represents the direction of in-plane magnetization in each image pixel. White arrows show the in-plane spin orientations in the DWs. Scale bar, 2 μm. ( c ) Sketch of right-handed Néel wall. ( d ) Histogram of angle α in DW boundary counted pixel-by-pixel in b shows a Gaussian distribution peaked at 180°, which corresponds to right-handed Néel wall. Inset shows the definition of the angle α , where n is a unit vector perpendicular to the domain boundary and always points from black domain to grey domain, m is the in-plane direction of the magnetization within the DW. ( e ) Monte Carlo simulation result of perpendicular magnetized film with the DMI shows right-handed chiral Néel walls with similar spin structures as seen experimentally in b . Full size image To be more quantitative, one can determine the statistical distribution of the magnetization direction within the DWs. We define the angle α ( Fig. 1d , inset) between the magnetization vector in the centre of the DW and the normal vector of the DW, and we measure the value of α pixel-by-pixel along the centre line of the DWs (Methods). The histogram plotted in Fig. 1d clearly shows that the angle α is scattered about a narrow distribution centred near 180°, which underscores that the DW is Néel type with right-handed chirality. The role of the DMI in stabilizing the chiral Néel wall structures observed in this system can be clarified by performing Monte Carlo simulations [31] , [32] , which predict right-handed chiral Néel walls as shown in the computed magnetization pattern reproduced in Fig. 1e . We also observed right-handed chiral Néel wall in [Ni/Co] n multilayers, where the first Co layer contacts the Pt(111) substrate. However, in those samples the domain size is very small, which makes measurement and analysis challenging. The larger domain size we find in [Co/Ni] n multilayers, where the first Ni layer contacts the Pt(111) substrate, results in better visibility of spin textures, and in this paper we focus on this class of multilayers. In layered structures made of high-symmetry (cubic or hexagonal) materials, the DMI arises only as an interface/surface effect [7] , [13] , [14] , [15] , [16] . This raises the question which interfaces/surfaces contribute to the DMI in our system. Interestingly, when we epitaxially grow identical [Co/Ni] n multilayers on an Ir(111) substrate instead of on a Pt(111) substrate, we find that the magnetization within DWs is no longer pointed from grey domains (+ M z ) to black domains (− M z ) but, instead, DW magnetization points in the opposite direction: from black domains to grey domains ( Fig. 2a ). This indicates left-handed chiral Néel walls [7] , [30] in [Co/Ni] n /Ir(111). Taken together, these results point to the importance of the interface between the substrate and the magnetic multilayer stacks in dominating the value of the DMI and governing the chirality of the DWs, with Ni/Pt(111) interfaces inducing right-handed chirality and Ni/Ir(111) inducing left-handed chirality. 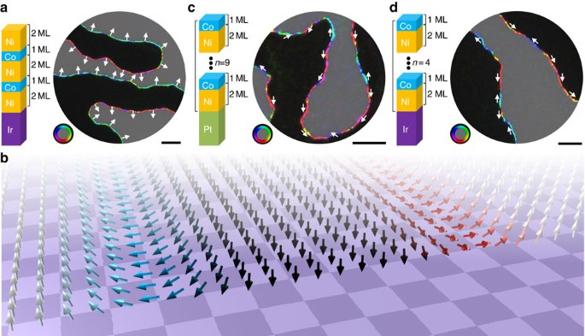Figure 2: The dependence of the DW chirality on substrates and thickness of films. (a) Compound SPLEEM images of Ni/[Co/Ni]2/Ir(111). Scale bar, 2 μm. (b) Sketch of left-handed Néel wall. (c) Compound SPLEEM images of [Co/Ni]9/Pt(111). Scale bar, 1 μm. (d) Compound SPLEEM images of [Co/Ni]4/Ir(111). Scale bar, 1 μm. Sketches on left sides in panelsa,canddshow multilayer structures of the samples. The colour wheel represents the direction of the in-plane magnetization. White arrows in the SPLEEM images additionally highlight the in-plane spin orientations inside the DWs. Figure 2: The dependence of the DW chirality on substrates and thickness of films. ( a ) Compound SPLEEM images of Ni/[Co/Ni] 2 /Ir(111). Scale bar, 2 μm. ( b ) Sketch of left-handed Néel wall. ( c ) Compound SPLEEM images of [Co/Ni] 9 /Pt(111). Scale bar, 1 μm. ( d ) Compound SPLEEM images of [Co/Ni] 4 /Ir(111). Scale bar, 1 μm. Sketches on left sides in panels a , c and d show multilayer structures of the samples. The colour wheel represents the direction of the in-plane magnetization. White arrows in the SPLEEM images additionally highlight the in-plane spin orientations inside the DWs. Full size image Estimating the strength of the DMI The interfacial origin of the DMI suggests that its value should be independent of the thickness of the stack. The contribution of the dipolar energy increases with the thickness of the multilayer stack and the dipolar force favours achiral Bloch walls. Therefore, a transition from chiral Néel walls to achiral Bloch walls can be expected above some thickness threshold [7] . Indeed, in the [Co/Ni] n /Pt(111) system, we observed achiral Bloch walls instead of chiral Néel walls when n ≥9 ( Fig. 2b ). Here the in-plane magnetization component of the DW randomly changes along each single DW, indicating absence of DW chirality. The observed DW spin structure transition can be used to quantify the strengths of the DMI at Ni/Pt(111) and Ni/Ir(111) interfaces. By calculating the energy of a Néel wall in [Co/Ni] 8 /Pt(111) and the energy of a Bloch wall in [Co/Ni] 9 /Pt(111), we bracket the strength of the DMI vector D ij at Ni/Pt(111) to be −1.05±0.18 meV per atom, where negative sign corresponds to right-handed chirality [30] . Analogous observations on the [Co/Ni] n /Ir(111) system show that the DW structure evolves to achiral Bloch-type DWs when n ≥4 ( Fig. 2c ), and we estimate the magnitude of D ij at Ni/Ir(111) to be+0.12±0.04 meV per atom [30] (Methods). Tailoring the chirality by interface engineering The experimental observation of opposite chirality at Ni/Pt(111) and Ni/Ir(111) interfaces raises the possibility to tailor chirality at an interface between Ni and a substrate composed of Ir and Pt in a tailored composition or structure. Following this idea, we inserted epitaxially grown Ir layers between Pt(111) substrates and [Co/Ni] n stacks. By tuning the thickness d Ir of Ir layers in the [Co/Ni] n /Ir/Pt(111) system, we observed that DW structure indeed transitions as a function of d Ir . Here we find three very different types of DW structures: right-handed chiral Néel walls for d Ir =0.6 atomic monolayer (ML; Fig. 3a ), achiral Bloch walls for d Ir =2.5 ML ( Fig. 3b ) and left-handed chiral Néel walls for d Ir =3 ML ( Fig. 3c ). To track this spin texture transition in more detail, we plot in Fig. 3d the histograms of the angle α as a function of d Ir , where we find a single peak near 180° (right-handed chiral Néel wall) for d Ir in the range of 0–1 ML, followed by a transition region between d Ir =1.5 and 2.5 ML, where two peaks in the histograms of the angle α are located at −90° and 90° (achiral Bloch walls). Increasing d Ir to 3 ML, the peak at −90° disappears and the other peak moves from 90° towards 0° (left-handed chirality), similar to the DW spin structure found when [Co/Ni] n multilayers are grown on bulk Ir. For a more quantitative discussion of the DW chirality and type, we first measure the magnetization direction at each pixel along the centre line of each DW, and then we define the asymmetry γ as γ =( N Left − N Right )/( N Left + N Right ), where N Left is the number of pixels one the DW where the magnetization points from the spin-down domain towards the spin-up domain and N Right is the number of DW pixels where the magnetization points from the spin-up domain towards the spin-down domain (a more detailed explanation of this process is described in Methods). We plot the dependence of asymmetry γ and peak positions on d Ir in Fig. 3e . With increasing d Ir , we find that γ changes gradually from −1 towards +1, whereas the fitted peak position evolves from 180° (right-handed) to 0° (left-handed). 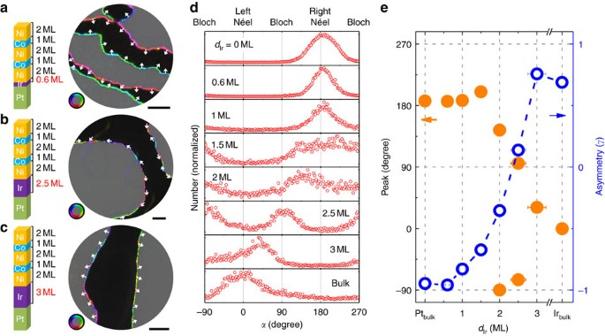Figure 3: Chirality as a function of Ir inserting layer thickness. (a–c) Compound SPLEEM images of Ni/[Co/Ni]2/Ir/Pt(111) with different thickness of the Ir layerdIr, (a) 0.6 ML, (b) 2.5 ML and (c) 3 ML. Scale bars, 1 μm. (d) Dependence of the histogram of the angleαondIrin the Ni/[Co/Ni]2/Ir/Pt(111) system. (e) Dependence of fitted peak position (left) and asymmetryγ(right) ondIrind; the asymmetryγquantifies chirality as −1 (right-handed), 0 (achiral) and 1 (left-handed). The error bars represent accuracy of Ir layer thickness (as derived from calibration of the Ir layer deposition rate). Figure 3: Chirality as a function of Ir inserting layer thickness. ( a – c ) Compound SPLEEM images of Ni/[Co/Ni] 2 /Ir/Pt(111) with different thickness of the Ir layer d Ir , ( a ) 0.6 ML, ( b ) 2.5 ML and ( c ) 3 ML. Scale bars, 1 μm. ( d ) Dependence of the histogram of the angle α on d Ir in the Ni/[Co/Ni] 2 /Ir/Pt(111) system. ( e ) Dependence of fitted peak position (left) and asymmetry γ (right) on d Ir in d ; the asymmetry γ quantifies chirality as −1 (right-handed), 0 (achiral) and 1 (left-handed). The error bars represent accuracy of Ir layer thickness (as derived from calibration of the Ir layer deposition rate). Full size image Phase diagram of chirality in [Co/Ni] n /Ir/Pt(111) We conclude from these observations that the DMI can be tuned by interface engineering. A phase diagram shown in Fig. 4a summarizes the dependence of DW chirality and type on the thickness of the magnetic multilayer stack (vertical axis) and d Ir (horizontal axis) in the [Co/Ni] n /Ir/Pt(111) system. Extending our procedure for estimating the strength of the DMI (Methods) to the phase diagram ( Fig. 4b ), we can track how the strength of the DMI gradually changes as a function of d Ir . Our results indicate that 3 ML Ir is sufficiently thick to fully quench the DMI between Ni and the Pt substrate and to fully develop the Ni/Ir interface DMI. Monte Carlo simulations can be used to compute a theoretical phase diagram ( Fig. 4c ). Here we represent the thickness of the magnetic multilayer by the strength of the dipole interaction D dipole , and the Ir spacer layer thickness d Ir by the magnitude and sign of D ij . The simulated phase diagram shows excellent agreement with the experimental phase diagram ( Fig. 4a ) when the D ij values used in the simulations correspond to the experimental values. The success of these simulations implies that a rich array of DW types and chirality might be achieved by extending materials choices beyond Ir/Pt(111) to generate different strengths and signs of the DMI. 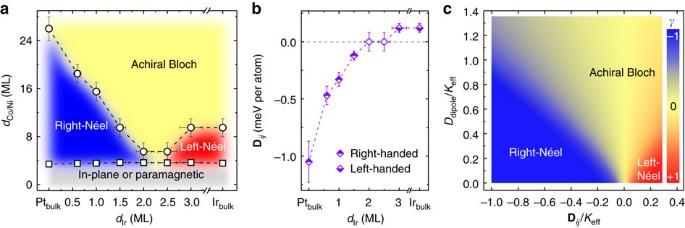Figure 4: Phase diagram of DW structure and estimated DMI. (a) Experimental DW type and chirality phase diagram of [Co/Ni]nmultilayer grown on Ir/Pt(111) substrate. The square dots indicate the transition from in-plane anisotropy to out-of-plane anisotropy, and circular dots indicate the transition from chiral Néel wall to achiral Bloch wall. The horizontal error bars represent accuracy of Ir layer thickness (as derived from calibration of the Ir layer deposition rate). Lower (upper) ends of vertical error bars represent experimental observations of Néel (Bloch) walls. The labels in-plane or paramagnetic refer to in-plane anisotropy or paramagnetic region where no out-of-plane magnetic contrast was observed. (b) Estimated strength of the DMI vectorDijdeduced from the data (circles) plotted ina. (c) Simulated phase diagram of DW chirality (asymmetryγ) by Monte Carlo simulation,Ddipolecorresponds to the strength of dipole interaction,Keffcorresponds to the effective magnetic anisotropy. Figure 4: Phase diagram of DW structure and estimated DMI. ( a ) Experimental DW type and chirality phase diagram of [Co/Ni] n multilayer grown on Ir/Pt(111) substrate. The square dots indicate the transition from in-plane anisotropy to out-of-plane anisotropy, and circular dots indicate the transition from chiral Néel wall to achiral Bloch wall. The horizontal error bars represent accuracy of Ir layer thickness (as derived from calibration of the Ir layer deposition rate). Lower (upper) ends of vertical error bars represent experimental observations of Néel (Bloch) walls. The labels in-plane or paramagnetic refer to in-plane anisotropy or paramagnetic region where no out-of-plane magnetic contrast was observed. ( b ) Estimated strength of the DMI vector D ij deduced from the data (circles) plotted in a . ( c ) Simulated phase diagram of DW chirality (asymmetry γ ) by Monte Carlo simulation, D dipole corresponds to the strength of dipole interaction, K eff corresponds to the effective magnetic anisotropy. Full size image The physics of the DW spin structure transitions might be associated with several possible mechanisms. One conjecture might invoke competition between right-handed DMI induced at Ni/Pt(111) interface regions and left-handed DMI induced at Ni/Ir(111) interface regions, which may happen when the Pt surface is not fully covered by the Ir thin film. Another possibility is that the Pt substrate may hybridize the electronic structure at the Ni/Ir interface through 1–3 ML Ir layer. This might affect chirality, as the D ij vector is related to both the electronic structure and to the spin-orbit coupling [5] . In addition, films and multilayers grown in (111) texture often have low-energy stacking faults; as a result, the crystal structure of such films can be fcc or hcp or a mixture, which may affect the value of the DMI. Additional very interesting research will be required to explore the physics of the observed possibility to tune chirality. We also notice that the strength of the DMI is very sensitive to subtle modifications of the film thickness in sputtered multilayers [8] , and we expect that the possibility of chirality tuning can be extended to sputtered films [8] , [9] , [33] . Our experimental results confirm that homochiral Néel wall structures are stable in a class of perpendicularly magnetized [Co/Ni] n multilayers in contact with Pt and Ir. Moreover, these experiments demonstrate that interface engineering provides a way to tailor the strength and the sign of the DMI and, as a result, to control DW spin structure in magnetic materials. Being able to manipulate DW chirality and spin texture points to rich possibilities to influence the dynamic properties of DWs through the DMI [4] , [5] , [7] , [13] , [14] , [15] , [16] , [34] , spin Hall effects [8] , [9] , [12] , [33] , [35] or Rashba effects [12] , [33] , [36] , [37] , thus presenting new opportunities for the design of high efficient spintronics devices. Real-space imaging The experiments were performed in the SPLEEM system at the National Center for Electron Microscopy at Lawrence Berkeley National Laboratory. With this instrument, magnetic contrast along two in-plane axes ( x and y ) and along the out-of-plane direction ( z ) can be mapped independently with lateral resolution of the order of 10 nm so that the three magnetic components M x , M y and M z of the spin structure inside the DWs can be resolved in real space. To maximize the magnetic contrast, 5 eV energy of the incident electron beam was chosen for both Co and Ni films. Supplementary Fig. S1 shows how SPLEEM imaging can be used to measure the DW structure in a [Co/Ni] n multilayer stack grown on Pt(111). The image reproduced in Supplementary Fig. S1a was acquired with the illuminating electron beam polarized along the surface normal direction and the strong black/white contrast results from the perpendicular magnetic anisotropy of the system. Using an in-plane polarized illumination electron beam, the in-plane components of the magnetization are imaged in Supplementary Fig. S1b,c : black/white contrast only appears in narrow bands and comparison with Supplementary Fig. S1a shows that these bands are at the DWs. Taken together, the three images, Supplementary Fig. S1a–c , reveal the orientation of the magnetization vector within this field of view: in Supplementary Fig. S1e , in-plane components of DWs are highlighted in colour as indicated by a colour wheel (inset) and the perpendicular magnetization component is shown by black (− M z ) and grey (+ M z ). The estimated DW width is ~150 nm, which is wider than what has been observed in other perpendicularly magnetized systems [38] . Our system as imaged in Supplementary Fig. S1 is close to a spin reorientation transition where the perpendicular anisotropy is weak [39] ; hence, it is reasonable to attribute the relatively large DW width to the well-known dependence of the DW width on the magnetic anisotropy [38] . Analysis of chirality An object is chiral if it cannot be mapped to its mirror image by rotations and translations alone. Examples of three-dimensional chiral structures include helical spin spirals and skyrmions. The spin structures of cycloidal spin spirals or Néel walls are two-dimensional examples. When the term chirality is used to refer rotational symmetry breaking for cycloidal spin spirals (or Néel walls with perpendicular anisotropy), then the usual definition can be ambiguous because after in-plane rotation such two-dimensional structures can be identical to their mirror image. However, the words ‘chirality’ or ‘handedness’ have been widely used to refer to this type of rotational symmetry breaking in cycloidal spin spirals. The analysis of chirality was done in three steps: (i) for each pixel along the centre line of each DW, the DW tangential direction and a normal vector n pointing from spin-down to spin-up (dark to bright) domains was determined (see inset in Fig. 1d ). This geometric information was derived from the magnetic domain patterns seen in the out-of-plane magnetization SPLEEM images. (ii) To determine the in-plane magnetization direction m at each pixel along the DW centre lines, we first averaged the grey values of the centred pixels and their eight nearest neighbour pixels in the two in-plane magnetization SPLEEM images. Then we find the in-plane magnetization direction m by comparing these averaged grey values from the in-plane images. Finally, we compute the angle α between m and n for every pixel on the DW. These angles between the geometric normal to the DW and the magnetization direction are plotted in the histograms in Figs 1d and 3d . (iii) To get a value for the degree of chirality, we define the asymmetry γ as γ =( N Left − N Right )/( N Left + N Right ), where N Left is the number of pixels one the DW in which α is between −90° and 90° (pointing from the spin-down domain towards the spin-up domain) and N Right is the number of DW pixels where α is between 90° and 270° (pointing from the spin-up domain towards the spin-down domain). In addition, the histograms in Fig. 3d were fitted by one or two Gauss curves. The position of the peaks in Fig. 3e indicates the average angle of the magnetization on the DW with respect to the orientation of the wall. Sample growth Pt(111) and Ir(111) substrates were cleaned by Ar + sputtering at 1.0 keV, followed by annealing at 850 °C in 3 × 10 −8 torr O 2 and final annealing at 1,100 °C for Pt(111) and 1,250 °C for Ir(111) under ultrahigh vacuum. Co, Ni and Ir layers were grown at 300 K by electron beam evaporations. Film thickness was calibrated by monitoring image intensity oscillations associated with atomic layer-by-layer growth. Ir thickness-dependent low-energy electron diffraction patterns show sharp spots for Ir insert layer grown on Pt(111) for d Ir =1, 2 and 3 ML, suggesting high-quality single crystalline Ir films. Estimation of the DMI strength To estimate the strength of the DMI vector D ij , we focus on the thickness-dependent measurement shown in Fig. 2 , where DWs changed from Néel walls to Bloch walls with increasing layer thickness. The free energy of Néel walls can be written as , where E EX corresponds to exchange energy, corresponds to the dipole energy of the Néel wall, E A corresponds to the magnetic anisotropy energy E A and corresponds to the DMI energy of the Néel wall. The free energy of Bloch walls is , where corresponds to dipole energy of Bloch wall and corresponds to the DMI energy of a Bloch wall. Here E EX and E A are equal for Néel wall and Bloch wall, and is higher than . For the [Co/Ni] n /Ir/Pt(111) case, D ij is always orthogonal to the vector ( S i × S j ), consequently the magnitude of the DMI for Bloch wall vanishes; thus, . Therefore, we can define an energy difference and such that when Néel walls are observed, and when Bloch walls are observed. By calculating the dipolar energy difference for Néel walls, , and for Bloch walls, , it is possible to estimate the magnitude of the DMI vector D ij in magnetic thin films [7] . Our model to calculate the dipolar energy difference is described in more detail in ref. 7 . In the calculation, the DW width is chosen as 150 nm, consistent with estimates of both Néel walls and Bloch walls observed in the SPLEEM images. The dipolar energy constant D dip is in the [Co/Ni] n case [7] , [39] , where μ 0 =4 π × 10 −7 H·m −1 , μ B =9.274 × 10 −24 A m 2 , μ Co =1.7 μ B , μ Ni =0.6 μ B , a || =2.49 Å. On the basis of Fig. 4a , we calculate the dipolar energy difference and of [Co/Ni] n /Ir/Pt(111) system numerically using the Matlab software [7] . The calculated dipolar energy difference and are summarized in Supplementary Table S1 . To check how robust these estimates might be with regard to assumptions of our model, we recalculated the energies as a function of varying DW width from 110 to 190 nm, and we found that only changes by 1%. Finally, we estimate the strength of the DMI vector as follows. For a square lattice, (refs 7 , 30 ) across one DW; this value changes to for a hexagonal lattice, independent of DW shape. The energy of the DMI is , where D DM is the strength of the DMI vector D ij . We know ; thus, the range of can be estimated based on the values listed in Supplementary Table S1 . (In the convention used here, right-handed/left-handed chirality corresponds to negative/positive DMI [30] ). Estimated D DM values are summarized in Supplementary Table S1 . Monte Carlo simulation The Monte Carlo simulations were carried out using the two-dimensional model described in refs 7 , 31 , 32 , where exchange interaction, magnetic anisotropy, dipolar interaction as well as DMI are considered. The total energy can be expressed as where S i and S j are spin moments located on atomic sites i and j in a two-dimensional plane, r i and r j are the position vectors of the atoms in sites i and j , J , K and D dip correspond to exchange energy, uniaxial out-of-plane anisotropy and dipole interaction, respectively, and H is an external magnetic field. The exchange interaction and the DMI are considered only among nearest neighbouring sites and vanish for larger distances, whereas dipole interactions involve all sites in the simulation. More details can be found in refs 7 , 31 . For fcc(111) interfaces/surfaces, the D ij vector is perpendicular to the distance vector R ij = R i − R j between i and j sites [40] . To capture the symmetry of fcc(111) interfaces/surfaces, our model introduces D ij vectors for each of the six neighbouring atoms surrounding an atom in a hexagonal lattice. Using D ij vectors as sketched in Supplementary Fig. S2 , Monte Carlo simulation predicts right-handed chiral DWs, as shown in the Fig. 1e . Simulations also indicate that the handedness of chiral DWs depends on the sign of the DMI vector D ij . To compute the simulated phase diagram ( Fig. 4c ), we set up starting spin arrays composed of two domains (magnetized up and down), separated by a DW in which starting spins are oriented in random directions. Subsequently, annealing these configurations allows us to find the energy ground state DW structures. The DW configurations were simulated as a function of D dip and D ij . In the figure, D dip and D ij were rescaled to D dip / K eff and D ij / K eff . How to cite this article: Chen, G. et al . Tailoring the chirality of magnetic domain walls by interface engineering. Nat. Commun. 4:2671 doi: 10.1038/ncomms3671 (2013).